The transcriptional regulator BBX24 impairs DELLA activity to promote shade avoidance inArabidopsis thaliana In response to canopy shade, plant vegetative structures elongate to gain access to light. However, the mechanism that allows a plastic transcriptional response to canopy shade light is not fully elucidated. Here we propose that the activity of PIF4, a key transcription factor in the shade signalling network, is modulated by the interplay between the BBX24 transcriptional regulator and DELLA proteins, which are negative regulators of the gibberellin (GA) signalling pathway. We show that GA-related targets are enriched among genes responsive to BBX24 under shade and that the shade-response defect in bbx24 mutants is rescued by a GA treatment that promotes DELLA degradation. BBX24 physically interacts with DELLA proteins and alleviates DELLA-mediated repression of PIF4 activity. The proposed molecular mechanism provides reversible regulation of the activity of a key transcription factor that may prove especially relevant under fluctuating light conditions. Light is a highly heterogeneous environmental factor controlling plant growth and survival, and defines the competitive relationships within the plant community [1] . Contrasting light gradients occur in plant canopies, so all plants are exposed to at least some degree of shade during their lifetime. Sun plants have evolved complex signalling mechanims to avoid shade through the promotion of developmental responses known as the shade-avoidance syndrome (SAS) that includes, among other responses, hypocotyl and petiole elongation, the upward orientation of leaves and the reduction of branching [2] . The relevance and the plasticity of this adaptive response are illustrated by the huge genetic variation that is found in nature [3] , [4] , [5] , [6] . The canopy light is rich in far-red (FR) and poor in red (R) and blue light. Shade-avoiding species have developed a precise machinery to finely perceive changes in R:FR ratio through the R/FR-light-absorbing phytochrome family of photoreceptors [2] . In open-light environments, when the R:FR ratio is high, the red-absorbing cytosolic form of phytochrome B, (phyB; Pr, max. absorbance=660 nm) is excited and photoconverted to a FR-absorbing form (Pfr, max. absorbance=730 nm) that moves to the nucleus, where it physically interacts with basic helix-loop-helix (bHLH) transcription factors called PHYTOCHROME-INTERACTING FACTORS (PIFs). Rapid phosphorylation and degradation of PIFs induces a dramatic reduction of growth rate in hypocotyls, stems and petioles [7] . In contrast, in shaded environments, the R:FR ratio is low and consequently the phytochromes are converted to the Pr form with low affinity for PIFs and preferential accumulation in the cytosol, allowing these transcription factors to accumulate and bind the promoters of cell elongation genes [8] . Transcriptional regulation in response to shade is not only regulated by PIFs. In fact, a small network of transcription factors, including the non-DNA-binding bHLHs LONG HYPOCOTYL IN FR LIGHT (HFR1), PHYTOCHROME RAPIDLY REGULATED1 (PAR1) and PAR2 modulate this process preventing an exaggerated shade-avoidance response by forming inactive heterodimers with PIFs [9] , [10] , [11] . Furthermore, double B-Box (BBX) containing zinc-finger transcription factors perform contrasting roles in the shade-avoidance response [10] . For instance, BBX21/STH2 and BBX22/STH3 act as negative regulators, while BBX24/STO and BBX25/STH1 promote hypocotyl growth of Arabidopsis seedlings under shade [11] , [12] . Moreover, all BBX members studied so far are involved in the CONSTITUTIVE PHOTOMORPHOGENIC1 signalling pathway promoting the shade response [11] , [12] . Several hormones are also essential components in the response to shade, owing to their role as central players in the regulation of cell elongation. Auxin, gibberellins (GAs) and brassinosteroids promote elongation [2] . For instance, a low R:FR ratio enhances both GA biosynthesis and responsiveness in Arabidopsis , thereby promoting the expression of GA-related genes [13] , [14] . GA signalling proceeds through the promotion of the degradation of DELLA proteins, a small family of nuclear-localized transcriptional regulators that repress GA-responses, such as cell elongation. The molecular mechanism by which DELLAs regulate transcription is through the physical interaction with transcription factors, including PIFs [15] . In open environments, DELLAs accumulate and inactivate PIF4, thus preventing cell elongation [16] , [17] . In agreement with this, enhanced petiole elongation under shade is accompanied by DELLA degradation [18] . Under low R:FR, GA biosynthesis is enhanced by the upregulation of GA20ox and GA3ox expression in petioles of A. thaliana [14] and Rumex palustris [19] . However, despite the function of GA-regulating cell elongation responses is well established, the GA signalling pathway operating under shade is uncertain [20] . Despite the importance of BBX proteins in the SAS [10] , the molecular mechanism by which BBX proteins exert their action under shade also remains to be determined. Here, we demonstrate that BBX24 is involved in the GA-branch promoting cell elongation under shade. In particular, our results show that BBX24 physically interacts with, and inactivates, DELLA proteins, thereby providing a flexible mechanism that explains the positive role of BBX24 in the control of shade-elongation responses. BBX24 regulates hormone-related genes in response to shade To determine the relative importance of BBX24 in the SAS, we examined the hypocotyl elongation when bbx24 and BBX24 -overexpressing ( BBX24ox ) seedlings were grown under white light (high R:FR) and simulated shade (low R:FR). Two bbx24 mutant alleles conferred normal hypocotyl elongation under high R:FR, but this ability was significantly reduced under low R:FR ( Fig. 1 ). In addition, hypocotyls were longer in BBX24ox seedlings than in the wild type under high and low R:FR, but still responded to simulated shade ( Fig. 1 ). These results demonstrate that BBX24 promotes hypocotyl elongation, but also other molecular elements are needed for a full response to shade. In fact, BBX25, its homologue, is one of these additional elements acting in parallel to BBX24. Although the bbx25-2 allele did not show defects in response to low R:FR, the bbx24-1 bbx25-2 double mutant displayed a greater reduction of the elongation response than each of the single mutants ( Fig. 1 ). Furthermore, a simulated canopy treatment that reduces both the irradiation and R/FR significantly altered the bbx25 seedling phenotype that failed to fully respond ( Supplementary Fig. 1 ). Again, the bbx25 allele was able to enhance the impaired phenotype of bbx24 in the double mutant ( Supplementary Fig. 1 ). 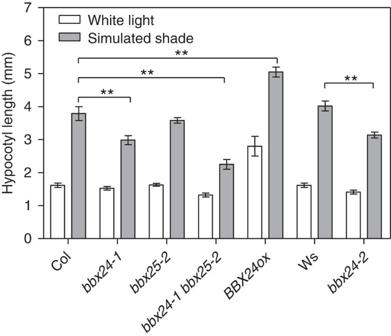Figure 1: Hypocotyl length in wild-type (Col-0 and Ws). bbx24andbbx25single and double mutants andBBX24oxseedlings grown under white light or simulated shade (high and low R:FR ratios, respectively) in a chamber for 5 days. Bars indicate mean±sem (n=20). **indicate differences between indicated means withP≤0.01 by Student'sttest. Figure 1: Hypocotyl length in wild-type (Col-0 and Ws). bbx24 and bbx25 single and double mutants and BBX24ox seedlings grown under white light or simulated shade (high and low R:FR ratios, respectively) in a chamber for 5 days. Bars indicate mean±sem ( n =20). **indicate differences between indicated means with P ≤0.01 by Student's t test. Full size image To identify genes regulated by BBX24 under simulated shade, we compared the transcriptomes of wild-type and bbx24-1 seedlings exposed to high or low R:FR. We set a false-discovery rate of 4.12% and 1.5-fold change as cutoff to select genes putatively regulated by BBX24. Among a total of 432 genes, 49 were misregulated independently of the light quality (that is, genotype effect), 84 genes were differentially expressed in the bbx24 mutant under high R:FR, and 299 genes were significantly altered under low R:FR (shade-regulated genes; Fig. 2a and Supplementary Data 1 ). The group of shade-regulated genes was enriched in gene categories associated with stress responses, cell-wall activity, secondary metabolism, hormone metabolism and transport-activity functions ( Fig. 2b ). D-chip analysis shows that shade-regulated genes can be clustered by transcription factors, signalling and hormone elements ( Fig. 2c ). Given that BBX proteins have been reported to regulate transcription through the interaction with DNA-binding transcription factors [12] , [21] , [22] , we searched for common regulatory motifs in the promoters of the shade-regulated genes that could indicate BBX24 partners in this process ( Supplementary Data 2 ). Among 299 genes regulated by BBX24 under simulated shade, we found that 212 genes (71%) contained one or two GA-response elements (125 and 87, respectively), and 77 genes (26%) contained auxin-response elements. Additionally, I-Box, G-Box, CCA1 and SORLIP1 elements were enriched (24, 23, 19, and 15% respectively; Supplementary Data 2 ). The link between BBX24 and hormone target genes under shade is also supported by the over-representation of auxin signalling genes previously linked to SAS, such as IAA29 and SAUR68 ( Supplementary Fig. S2 and Supplementary Data 1 ). Auxin conjugation ( GH3.3 ), GA catabolism ( GA2ox1, GA2ox2 ), ethylene synthesis ( ACS2 ) and circadian clock ( ELF4 ) genes were also regulated by BBX24 under shade ( Supplementary Fig. 2 ). Interestingly, GA20ox2 and GA3ox1 genes that are required for the synthesis of active GAs do not belong to the group of BBX24 shade-regulated genes ( Supplementary Data 2 ), but their expression in bbx24 seedlings exposed to shade is significantly different to wild type by quantitative reverse-transcription–PCR (RT-qPCR) analysis ( Supplementary Fig. 2 ). In summary, the global expression analysis suggests that BBX24 can act directly or indirectly in conjunction with hormonal and light/circadian clock networks to promote hypocotyl elongation under shade. 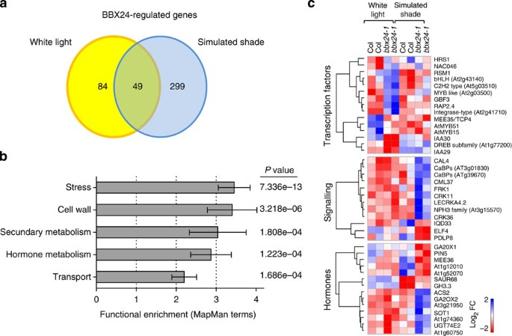Figure 2: BBX24 regulates 299 genes under shade. (a) Venn diagram showing the number of genes regulated by BBX24 under white light and shade. (b) Functional classification of the 299 genes regulated by BBX24 under shade. A bootstrap analysis was done to estimate the over-representation of each functional class and error bars, and thePvalues are indicated. (c) Cluster analysis of BBX24-regulated genes under shade using the D-chip program: transcription factors, signaling and hormone metabolism categories are shown. Figure 2: BBX24 regulates 299 genes under shade. ( a ) Venn diagram showing the number of genes regulated by BBX24 under white light and shade. ( b ) Functional classification of the 299 genes regulated by BBX24 under shade. A bootstrap analysis was done to estimate the over-representation of each functional class and error bars, and the P values are indicated. ( c ) Cluster analysis of BBX24-regulated genes under shade using the D-chip program: transcription factors, signaling and hormone metabolism categories are shown. Full size image GAs restore elongation of bbx24 hypocotyls under shade Enhanced production of active auxins and GAs is required for proper hypocotyl growth in response to low R:FR [18] , [23] . As a significant proportion of genes regulated by BBX24 under low R:FR belong to the auxin and GA pathways ( Fig. 2 and Supplementary Fig. 2 , Supplementary Data 1 and 2 ), we examined the effects of hormone levels to evaluate which of them is responsible for the bbx24 phenotype. Picloram, a synthetic auxin (0.5 or 1 μM), was equally effective in promoting hypocotyl elongation in wild-type and in bbx24 mutant seedlings ( Fig. 3a and Supplementary Fig. 3 ). In a complementary manner, 1-N-naphthylphthalamic acid (NPA, 0.5 μM), an inhibitor of polar-auxin transport, treatment reduced the elongation in wild-type and bbx24 seedlings under high and low R:FR, indicating the shade response similar between both genotypes ( Fig. 3a and Supplementary Fig. 4 ). Other hormones involved in promoting hypocotyl elongation in the SAS, such as ethylene and brassinosteroids [23] , [24] , did not rescue the mutant phenotype of bbx24-1 and bbx24-2 seedlings under low R:FR ( Supplementary Fig. 3 ). 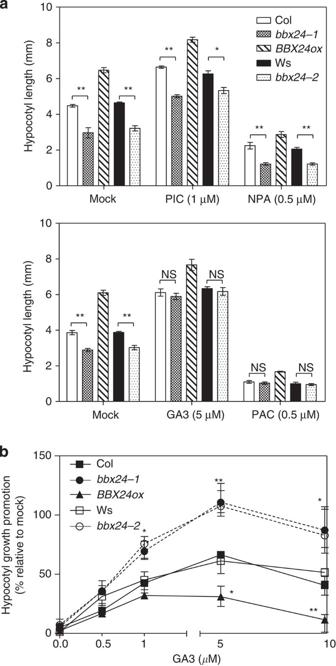Figure 3: Gibberellins (GAs) restore hypocotyl length ofbbx24seedlings under shade. (a) GA3, but not picloram (auxin), restores the hypocotyl length ofbbx24mutant seedlings under shade. paclobutrazol (PAC; GA synthesis inhibitor), but not 1-N-naphthylphthalamic acid (NPA; auxin transport inhibitor), suppresses the hypocotyl elongation mediated by BBX24 under shade. (b) GA3dose-response curve for hypocotyl growth promotion relative to mock (%) in wild-type, twobbx24mutant alleles andBBX24oxtransgenic lines. Bars inaand points inbindicate means±s.e.m. (n=20). *P≤0.05 and **P≤0.01 by Student’st-test. NS, not significant differences between indicated means. Figure 3: Gibberellins (GAs) restore hypocotyl length of bbx24 seedlings under shade. ( a ) GA 3 , but not picloram (auxin), restores the hypocotyl length of bbx24 mutant seedlings under shade. paclobutrazol (PAC; GA synthesis inhibitor), but not 1-N-naphthylphthalamic acid (NPA; auxin transport inhibitor), suppresses the hypocotyl elongation mediated by BBX24 under shade. ( b ) GA 3 dose-response curve for hypocotyl growth promotion relative to mock (%) in wild-type, two bbx24 mutant alleles and BBX24ox transgenic lines. Bars in a and points in b indicate means±s.e.m. ( n =20). * P ≤0.05 and ** P ≤0.01 by Student’s t -test. NS, not significant differences between indicated means. Full size image Remarkably, we found that the defective hypocotyl elongation phenotype of bbx24-1 and bbx24-2 seedlings under shade was fully rescued by the addition of GA 3 ( Fig. 3a ). To further support the functional relationship between BBX24 and the GA pathway, we performed a GA 3 dose-curve response ( Fig. 3b ). bbx24-1 and bbx24-2 seedlings were hypersensitive to GA 3 and showed significant differences compared with the wild type at 1 μM that further increased at 5 μM. In contrast, BBX24 ox seedlings showed less sensitivity to the exogenous application of GA 3 than the wild type. These results suggest that BBX24 is involved in the regulation of GA metabolism and/or signalling under shade. BBX24 promotes shade avoidance through PIF4 PIF4 is a central component of the transcriptional network regulating growth and it integrates diverse signals, including light and GAs [16] , [17] . Furthermore, PIF4 promotes SAS through binding to the G-box (CACGTG) in the promoter of shade genes [9] . Interestingly, promoters of BBX24-regulated genes are enriched in the same cis -element ( Supplementary Data 2 ). Then, we hypothesized that BBX24 is implicated in the PIF4-dependent shade signalling. To have a better understanding of this possible functional connection we generated bbx24 pif4 double mutant. Hypocotyls of pif4, bbx24 and pif4 bbx24 mutants were very similar to each other and shorter than the wild type under low R:FR ( Fig. 4a ). Furthermore, we compared the Arabidopsis transcriptomes regulated by BBX24 (our data), PIF4 and PIF7 when seedlings were grown under low R:FR [25] , [26] , [27] . The meta-analysis of 299 BBX24-regulated and 246 PIF-regulated genes under shade found that 16 genes were co-regulated by BBX24 and PIFs ( Fig. 4b and Supplementary Data 3 ). We observed a significant and positive association between genes regulated by BBX24 and PIFs (representation factor=4.8, P <2.87e−0.7). These results suggest that BBX24 and PIF transcription factors are involved in the same signalling pathway and act in the same direction promoting elongation. Furthermore, we compared BBX24 shade-regulated genes with the PIF4 targets obtained by chromatin immunoprecipitation [28] . Remarkably, 27 genes (9%) are both bound in vivo by PIF4 and commonly regulated by both proteins ( Supplementary Data 4 ). By RT-qPCR analysis, we confirmed that the expression of genes upregulated by BBX24 under shade, IAA29 , SAUR68 and GH3.3 , are downregulated in bbx24, pif4 and bbx24 pif4 mutants in a similar manner. PIL1 , a gene not represented in the ATH1 chip, but known to be an early shade-regulated gene, also showed a reduced expression in single and double mutants of BBX24 and PIF4 ( Fig. 4c ). Conversely, plants overexpressing BBX24 showed an enhanced induction of IAA29 , SAUR68 and GH3.3 gene expression in response to shade ( Fig. 4c ). The results of both expression and physiological experiments suggest that BBX24 and PIF4 participate in the same signalling pathway co-regulating a common group of genes that promote elongation under shade. 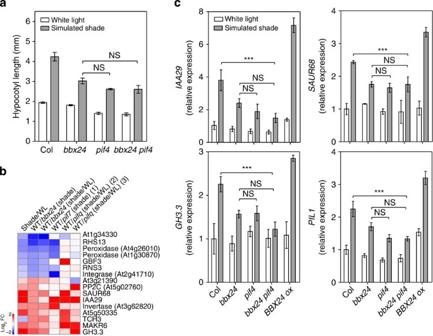Figure 4: BBX24 promotes shade avoidance through PIF4. (a) Hypocotyl length of wild-type,bbx24andpif4single and double mutant seedlings grown under white light and simulated shade. (b) Co-regulated genes by BBX24 (data of this work) and PIFs under shade (1) Liet al.25, (2) Leivaret al.27, (3) Hornitscheket al.26(c)IAA29, SAUR68, GH3.3andPIL1expression measured by RT-qPCR showing co-regulation by BBX24 and PIF4 under shade. The transcript levels were standardized to the wild type under white light. Bars inaandcindicate means±s.e.m. (n=20 andn=3, respectively). ***P≤0.001 by Student’st-test. NS, not significant differences between indicated means. Figure 4: BBX24 promotes shade avoidance through PIF4. ( a ) Hypocotyl length of wild-type, bbx24 and pif4 single and double mutant seedlings grown under white light and simulated shade. ( b ) Co-regulated genes by BBX24 (data of this work) and PIFs under shade (1) Li et al . [25] , (2) Leivar et al . [27] , (3) Hornitschek et al . [26] ( c ) IAA29, SAUR68, GH3.3 and PIL1 expression measured by RT-qPCR showing co-regulation by BBX24 and PIF4 under shade. The transcript levels were standardized to the wild type under white light. Bars in a and c indicate means±s.e.m. ( n =20 and n =3, respectively). *** P ≤0.001 by Student’s t -test. NS, not significant differences between indicated means. Full size image BBX24 interacts with DELLAs to relieve repression of PIF4 Previous evidence clearly demonstrate that much of the DELLAs’ involvement in the control of cell expansion is exerted through the modulation of PIFs’ activity [16] , [17] . The observations that the addition of GA3 in the growth medium recovers the bbx24 phenotype and the large overlap between PIF4 and BBX24 transcriptomes indirectly link BBX24 function to DELLA activity, Indeed, we found that this functional connection was correlated with the physical interaction between BBX24 and GAI and RGA, the two major DELLAs controlling hypocotyl elongation ( Fig. 5a ) [29] . The results of yeast-two-hybrid assays with truncated BBX24 protein did not identify any particular interacting domain, suggesting that BBX24 might establish several and independent contacts with M5-GAI ( Fig. 5b ). A similar analysis with deleted versions of GAI highlighted the importance of the leucine heptad repeat 1 ( Fig. 5b ) for the interaction, as reported for other partners [16] , [17] , [30] . Importantly, we also confirmed the interaction in plant cells. YFN-BBX24 and YFC-GAI interacted in nuclei of epidermal cells of Nicotiana benthamiana leaves as shown by means of bimolecular fluorescence complementation (BiFC) assays, whereas fluorescence in nuclei of control leaves co-expressing YFN-BBX24/YFC and YFN/YFC-GAI pairs was below detection limits ( Fig. 5c ). In addition, we confirmed this physical interaction by co-immunoprecipitation of BBX24-YFP and GAI-RFP transiently co-expressed in N. benthamiana leaves ( Fig. 4d , Supplementary Fig. 5 ). 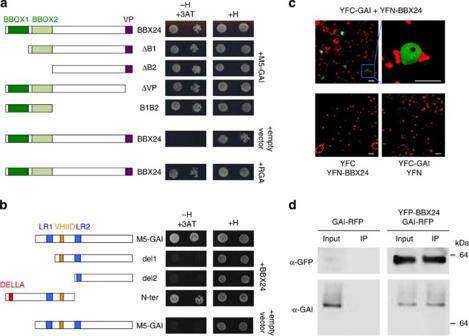Figure 5: BBX24 interacts physically with DELLAs. (a,b) Yeast-two-hybrid (Y2H) assay analysing the interaction between BBX24 and GAI and RGA. (c) Bimolecular Fluorescence Complementation (BiFC) analysis inN. benthamianaleaves of BBX24 and GAI fusions to N- and C-terminal fragments of YFP, respectively (upper photographs). Nuclei of control leaves co-expressing YFN-BBX24/YFC and YFN/YFC-GAI pairs are shown in the bottom photographs. Scale bars, 40 and 16 μm (d) Co-immunoprecipitation assay showing the interaction between BBX24 and GAI in leaves ofN. benthamiana. Figure 5: BBX24 interacts physically with DELLAs. ( a , b ) Yeast-two-hybrid (Y2H) assay analysing the interaction between BBX24 and GAI and RGA. ( c ) Bimolecular Fluorescence Complementation (BiFC) analysis in N. benthamiana leaves of BBX24 and GAI fusions to N- and C-terminal fragments of YFP, respectively (upper photographs). Nuclei of control leaves co-expressing YFN-BBX24/YFC and YFN/YFC-GAI pairs are shown in the bottom photographs. Scale bars, 40 and 16 μm ( d ) Co-immunoprecipitation assay showing the interaction between BBX24 and GAI in leaves of N. benthamiana. Full size image At least two possible mechanistic models based on the interaction between DELLAs and BBX24 could explain the positive role of BBX24 in the SAS: either BBX24 is a negative regulator of DELLA activity, thereby alleviating the repression of PIF4 by DELLAs, or alternatively, BBX24 is a co-activator of PIF4 that is negatively regulated by DELLAs. To distinguish between these two hypotheses, we set up a transient expression assay in N. benthamiana leaves using PIL1::LUC as a reporter for the activity of PIF4 (ref. 31 ), given that PIL1 is a direct target of transcriptional regulation by PIF4 (ref. 32 ), and importantly, is also regulated by BBX24 activity under shade ( Fig. 4c ). As expected, expression of PIF4 increased PIL1::LUC activity at least threefold with respect to basal levels, and this induction was strongly reverted by co-expression of GAI ( Fig. 6a ). Interestingly, PIF4 activity was not altered by co-expression of BBX24, ruling out that this protein acts as a direct co-regulator of PIF4 activity. However, co-expression of BBX24 alleviated the repression imposed by GAI upon PIF4 ( Fig. 6a ), suggesting that this could be the mechanism by which BBX24 promotes the transcriptional response to shade through PIF4. Indeed, competition for DELLAs by PIF4 and BBX24 was further supported by BiFC experiments in which the interaction between PIF4 and GAI was impaired by co-expression of BBX24 ( Fig. 6b ). 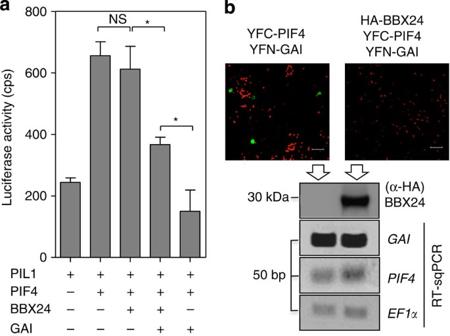Figure 6: BBX24-GAI protein interaction promotes PIF4 activity. (a) Transient expression assay inN. benthamianaleaves usingPIL1::LUCas a reporter (‘cps’ are the Firefly Luciferase (LUC) fluorescence ‘counts per sample’, relative to the control Renilla Luciferase fluorescence used to normalize agro infiltration. BBX24 expression alleviates the repression of PIF4 by GAI. Bars indicate means±s.e.m. (n=2 or 3). *P≤0.05 by Student’st-test, NS, not significant. (b) Bimolecular Fluorescence Complementation (BiFC) assay between PIF4 and GAI inN. benthamianaleaves is reverted by co-expression of BBX24. The bottom panels show thatBBX24, GAIandPIF4are expressed even if no BiFC signal is detected, according to the immunodetection of HA-BBX24 and semiquantitative PCR. Scale bars, 40 μm. Figure 6: BBX24-GAI protein interaction promotes PIF4 activity. ( a ) Transient expression assay in N. benthamiana leaves using PIL1::LUC as a reporter (‘cps’ are the Firefly Luciferase (LUC) fluorescence ‘counts per sample’, relative to the control Renilla Luciferase fluorescence used to normalize agro infiltration. BBX24 expression alleviates the repression of PIF4 by GAI. Bars indicate means±s.e.m. ( n =2 or 3). * P ≤0.05 by Student’s t -test, NS, not significant. ( b ) Bimolecular Fluorescence Complementation (BiFC) assay between PIF4 and GAI in N. benthamiana leaves is reverted by co-expression of BBX24. The bottom panels show that BBX24, GAI and PIF4 are expressed even if no BiFC signal is detected, according to the immunodetection of HA-BBX24 and semiquantitative PCR. Scale bars, 40 μm. Full size image To better understand the timing of BBX24-DELLA module action under shade, we measured the expression of some genes and DELLA protein levels in short-term shade. Seedlings of wild-type, bbx24 and BBX24ox were cultivated in white light for 5 days and then exposed between 0 and 2 h to supplemental FR at the end of the photoperiod. We found that PIL1, GH3.3 and SAUR68 were dramatically and rapidly upregulated by simulated shade in wild-type seedlings and the absence of BBX24 significantly reduced their expression ( Fig. 7a ). Furthermore, RGA protein levels were not altered in wild-type, bbx24 and BBX24ox seedlings cultivated for 2 h of short-term shade ( Fig. 7b , Supplementary Fig. 5 ). As predicted by our BBX24-DELLA interaction model, these results suggest that the expression of BBX24-regulated genes under shade may be altered rapidly without the need for degradation of RGA proteins, a process that requires more time for the action of proteosome. However, the transcript levels of RGA and PIF4 in short-term shade were not affected by the presence of BBX24 ( Supplementary Fig. 6 ), we found that long-term shade significantly increased the expression of DELLAs, PIF4 and PIL1 mediated by BBX24 ( Supplementary Fig. 7 ). 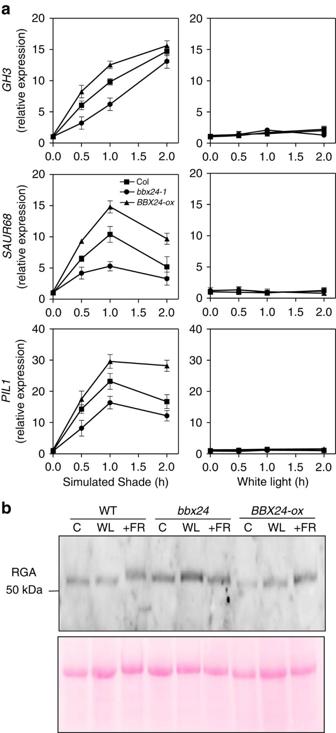Figure 7: Expression of shade-regulated genes and DELLA protein levels in short-term simulated shade. Seedlings of wild type,bbx24andBBX24oxwere cultivated in white light for 5 days and then exposed between 0 and 2 h to supplemental far-red (FR) at the end of the photoperiod. (a) Shade-regulated genes change dramatically in short-term shade. GH3.3, SAUR68andPIL1expression were measured by RT-qPCR at 0, 0.5, 1 and 2 h after exposing seedlings to simulated shade. The transcript levels were standardized to the wild type under white light. Means±s.e.m. (n=4). (b) RGA protein levels do not change in short-term shade in a western blot using anti-RGA antibody (1:300). C, control att=0 h; WL, white light att=2 h; +FR, simulated shade att=2 h. Figure 7: Expression of shade-regulated genes and DELLA protein levels in short-term simulated shade. Seedlings of wild type, bbx24 and BBX24ox were cultivated in white light for 5 days and then exposed between 0 and 2 h to supplemental far-red (FR) at the end of the photoperiod. ( a ) Shade-regulated genes change dramatically in short-term shade. G H3.3, SAUR68 and PIL1 expression were measured by RT-qPCR at 0, 0.5, 1 and 2 h after exposing seedlings to simulated shade. The transcript levels were standardized to the wild type under white light. Means±s.e.m. ( n =4). ( b ) RGA protein levels do not change in short-term shade in a western blot using anti-RGA antibody (1:300). C, control at t =0 h; WL, white light at t =2 h; +FR, simulated shade at t =2 h. Full size image Our model also predicts that enhanced accumulation of DELLA proteins should cause resistance to the overexpression of BBX24 under shade conditions. To test this possibility, we examined the phenotype of pGAI::gai-1D:GR (gai-1:GR) seedlings expressing a conditional allele of GAI resistant to GA-induced degradation fused to the rat glucocorticoid receptor (GR) under the control of the native GAI promoter [28] . The gai-1:GR fusion protein is retained in the cytoplasm in the absence of the added steroid dexamethasone (DEX), whereas application of DEX results in its relocation from the cytoplasm to the nucleus. In the absence of DEX, hypocotyls of gai-1 and gai-1:GR seedlings were shorter and similar to the wild-type seedlings under simulated shade, respectively ( Fig. 8 ); similarly, the gai-1:GR transgene did not alter the phenotype of BBX24ox seedlings under the same light conditions ( Fig. 8 ). As expected, DEX treatment caused an inhibition of hypocotyl growth under shade of gai-1:GR seedlings, which was then comparable with that of the gai -1 mutant; and this inhibition was even more evident in the BBX24ox background ( Fig. 8 ), indicating that the promotion of elongation by BBX24 under shade was in fact compromised by increasing DELLA’s levels. This result is therefore in agreement with DELLAs acting downstream of BBX24 in the shade response. 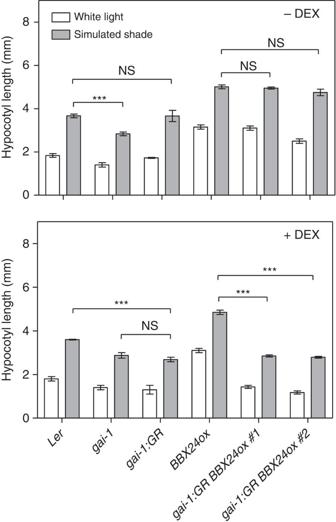Figure 8: Hypocotyl length of wild-type,gal-1,gal-1:GR,BBX24oxandgal-1:GR BBX24oxmutant seedlings grown under white light and simulated shade in response to application of the steroid dexamethasone (+DEX) or mock solution (−DEX). Bars indicate mean±s.e.m. (n=15). ***P≤0.001 by Student’st-test. NS, not significant differences between indicated means. Figure 8: Hypocotyl length of wild-type, gal-1 , gal-1:GR , BBX24ox and gal-1:GR BBX24ox mutant seedlings grown under white light and simulated shade in response to application of the steroid dexamethasone (+DEX) or mock solution (−DEX). Bars indicate mean±s.e.m. ( n =15). *** P ≤0.001 by Student’s t -test. NS, not significant differences between indicated means. Full size image An outstanding question in modern biology is how plants integrate environmental information in a plastic manner to modulate developmental habits. The evidence presented in this work provides a molecular mechanism that modulates the pathway linking the perception of shaded environments and the transcriptional regulation that ultimately results in a change in the growth pattern ( Fig. 9 ). The mechanism by which BBX24 regulates DELLA’s activity in the context of shade avoidance is physiologically relevant, as it illustrates how light quality signals may relay the information through protein–protein interaction originating a small transcriptional regulatory network with well-defined flexible properties allowing a rapid and reversible response to shade. We have provided clear evidence that bbx24 phenotype is rescued by GAs and operates in the GA signalling pathway by interrupting GAI-PIF4 interaction. In fact, we found that the impaired elongation phenotype of bbx24 mutants is rescued by the addition of GA, and also the bbx24 mutants are more sensitive to GA ( Fig. 3 ). Nevertheless, the expression of some metabolic GA genes, targets of DELLA regulation, did not explain the phenotype of bbx24 mutants. While GA20ox2 and also GA2ox2 were downregulated GA3ox1 and GA2ox1 were upregulated by shade in the bbx24 mutant ( Supplementary Fig. 2 ). These results suggest that the feedback regulation of GA metabolic genes by DELLAs involves unknown elements also affected by BBX24. In addition, our results provide a novel case in which DELLA activity is downregulated by a mechanism different to GA-induced protein degradation mediated by the GID1 receptors as was demonstrated before [33] . The results suggest that some DELLA repressors could be sequestered by BBX24 proteins which would allow more PIF transcription factors to activate cell growth to elongate vegetative structures avoiding light competition under shade. 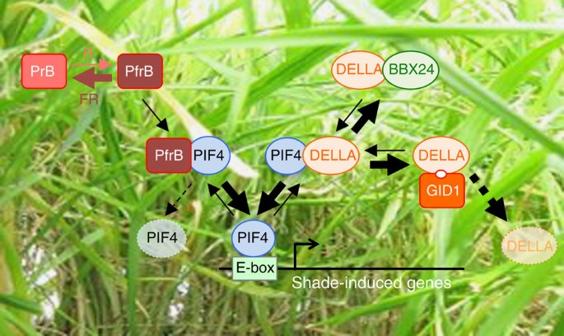Figure 9: Model of BBX24 action in shade signalling. In open environments with a high R:FR, the major form of phyB is PfrB, which destabilizes PIF4 and prevents the expression of shade-induced genes. In crowded stands with a low R:FR, the Pr form of phyB (PrB) increases and PIF4 binds to the G-box (CACGTG) in the promoter of genes that promote elongation. The PIF4 stability increases under shade because (i) PrB has low affinity to bind with PIF4 for degradation, (ii) PrB is mainly re-located to the cytosol, and (iii) BBX24 decreases the amount of DELLAs capable to interact with PIF4. We speculate that an early or intermittent response to shade favors protein–protein reversible interactions between DELLAs and BBX24, while a prolonged shade favors quantitatively the GA-induced irreversible degradation of DELLAs by the proteosome machinery. The thickness of the arrow indicates the reaction favoured under shade. Figure 9: Model of BBX24 action in shade signalling. In open environments with a high R:FR, the major form of phyB is PfrB, which destabilizes PIF4 and prevents the expression of shade-induced genes. In crowded stands with a low R:FR, the Pr form of phyB (PrB) increases and PIF4 binds to the G-box (CACGTG) in the promoter of genes that promote elongation. The PIF4 stability increases under shade because (i) PrB has low affinity to bind with PIF4 for degradation, (ii) PrB is mainly re-located to the cytosol, and (iii) BBX24 decreases the amount of DELLAs capable to interact with PIF4. We speculate that an early or intermittent response to shade favors protein–protein reversible interactions between DELLAs and BBX24, while a prolonged shade favors quantitatively the GA-induced irreversible degradation of DELLAs by the proteosome machinery. The thickness of the arrow indicates the reaction favoured under shade. Full size image Owing to their activity as negative regulators of an increasing number of DNA-binding transcription factors, DELLAs act as general growth repressors that need to be inactivated to promote cell expansion [15] , [34] , although it has also been shown that DELLAs can act as cofactors promoting the activity of some transcription factors [35] , [36] , [37] . Interestingly, all known environmental signals that promote growth induce the degradation of DELLA proteins by the proteosome. This is the case of higher ambient temperatures [38] , darkness periods [39] , [40] and also low R:FR ratios [18] , all of which presumably alter GA levels or the accumulation of GID1 receptors to drive to the reduction of DELLAs in the nucleus. However, the interaction of DELLA proteins with BBX24 represents an alternative mechanism for the modulation of DELLA activity that does not involve protein degradation, but allows the sequestration of DELLA protein in competition with the PIF4 transcription factor. This regulatory cascade based on protein–protein interactions ultimately regulating gene expression represents an emerging theme in plant signalling pathways. For instance, a triple HLH/bHLH cascade has been described by which the DNA-binding ability of a bHLH transcription factors (PIF4 or ACE1) is negatively regulated by the physical interaction with an HLH protein (HFR1, PAR1 or IBH1), which in turn is repressed by direct interaction with another HLH protein such as PRE1 (refs. 41 , 42 ). An equivalent regulatory module has been reported for MYC2, whose transcriptional activation capacity is repressed by interaction with the JAZ regulators, while DELLA proteins interact physically with JAZs to revert this repression [30] , [43] . BBX proteins have been previously defined as transcriptional regulators [12] , [21] , [22] with opposite regulating functions in shade and other developmental processes [10] . For example, BBX21 inhibits ABI5 expression by interfering with HY5, and also, ABI5 protein binding to the ABI5 gene promoter in germinating seeds [22] . Moreover, BBX24 and BBX25 interact with HY5 preventing its DNA-binding to the promoter of BBX22 gene to induce its expression in seedling de-etiolation [12] . In addition, BBX32 may interact physically with other BBX DNA-binding protein, like BBX21, and avoid the promotion of photomorphogenic genes [21] . In this context, our results show that BBX24 indirectly regulates the DNA-binding activity of PIF4 by the direct interference with DELLAs to promote cell elongation under shade. An additional property of the BBX24-DELLA-PIF4 regulatory module, particularly important in the context of shade avoidance, is the intrinsic reversibility conferred by protein–protein interactions, compared with cascades involving de novo protein synthesis, or protein degradation. This plasticity may become critical in short-term or transient exposure to shade. In fact, the capacity of perception and transduction of light gap signals in a dynamic canopy environment to adjust the growth of vegetative structures is relevant to define the competitive relationships between plant individuals. Albeit the importance of kinetics in the shade growth response in different species, the knowledge of molecular mechanisms involved in each phase of growth elongation is scarce [30] and limited to the upregulation of some genes like PIL1 , ATHB2 or HFR1 in short-term shade [11] , [44] . Here, we propose a possible mechanism for a reversible and a rapid response to shade that involves the protein–protein interaction between BBX24 and DELLAs that competes for the interaction between DELLAs and PIF4. One of the most important features inherent to the topology of the BBX24-DELLA-PIF4 module is that the transcriptional output of the cascade depends on the fine balance between molecular elements, which is determined by different and sometimes antagonistic signals that become integrated through protein–protein interactions. Given that DELLA and PIF4 levels are differentially influenced by temperature among other signals, and BBX24 and PIF4 stability has also been found to be dependent on light intensity, this regulatory module would render responses to shade in variable magnitudes depending on other environmental conditions and developmental phases. In fact, the shade-avoidance mechanisms may operate in different development processes including, between others, the control of seed germination, the orientation of branches and leaves, the elongation of stems, the production of new branches or tillers and the performance of the photosynthetic apparatus. Then, the capacity of plants to exploit rapid and efficiently the light opportunities in competition with neighbours would be a major determinant of evolutionary success. So it would be interesting to investigate if the molecular mechanism depicted here has been subject to adaptive pressure in different developmental situations and habitats. Plant material The mutants and transgenic lines used in this study have been described previously: bbx24-1, bbx25-2, bbx24-1 bbx25-2 and BBX24ox in Col background, and bbx24-2 in WS background [12] , [45] ; gai-1:GR lines [46] , and the PIF4ox line [17] . pif4-101 was obtained from the Arabidopsis Biological Resource Center. To generate HA-BBX24 fusion, the pENTR-BBX24 was recombined by LR reaction ( http://www.invitrogen.com ) with pEarleyGate-204 (ref. 47 ). gai-1:GR BBX24ox lines were generated by crossing HA-BBX24 with gai1:GR lines and selected for homozygous progeny by PCR using primers listed in Supplementary Table 1 . Growth conditions and light treatments In general we used the same experimental protocols described in Crocco et al . [11] Seeds were sown in clear plastic boxes on 0.8% agar/water, and incubated in darkness at 4 °C to reduce dormancy and homogenize germination. After 4 days, imbibed seeds were exposed to a red pulse and incubated in darkness for 24 h at 25 °C to induce germination. Then, the boxes with seedlings were transferred to white light for de-etiolation during 2 days. Three-day-old seedlings were exposed to white light or white light supplemented with FR lamps in a growth chamber at 22 °C settled with a short-day photoperiod (8 h light+16 h dark) for 5 days. White light treatment consisted in mercury lamps (General Electric HR175/R/DX/FL39 mercury 33026) that established a high R:FR=2,3. Simulated shade was generated with the addition of incandescent lamps (Philips, R19-100R20/FL/S) and two paolini filters with a red acetate (Paolini 2031; La Casa del Acetato, Buenos Aires, Argentina) placed laterally into the growth chamber that established a low R:FR=0.35. The up radiation was similar for both light treatments (PAR=100 μmol m −2 s −1 ). In addition, we used a simulated canopy condition that reduces both irradiance and R/FR ratio (PAR=30 μmol m −2 s −1 and R:FR=0.30) by putting one paolini filter on the top of the boxes with seedlings. Spectral photon fluencies were estimated with a Li-Cor (Li-188B, LiCor Corp., Lincoln, NE, USA), and PAR and R:FR were measured using an SpectroSense2 attached with a SKR-1850SS2 light sensor (Skye Instruments Ltd., Powys, UK). Hormone experiments Seeds were sown in agar/water medium supplemented with synthetic hormones: indole-3-acetic acid, GA 3 , precursor of ethylene (ACC) or brassinosteroids (EpiBL); or specific inhibitors: NPA and paclobutrazol (PAC) that inhibit the auxin polar transport and the endogenous GA synthesis, respectively. For DEX experiment, seeds were sown in agar/water on a filter paper. The experimental protocol was similar to those exposed before with little adjustments. To allow germination during PAC treatments, seeds were first sown and germinated for 24 h under white light on top of a wet filter paper, after which the filter paper was transferred to the MS plate containing PAC at the indicated concentrations. In the DEX experiments, 2 μM DEX (+DEX) or control solution with ethanol (−DEX) was added on the top of filter papers immediately before to start the light treatments. RT-qPCR experiments For RNA expression, 100 mg of fresh seedlings were harvested and frozen immediately in liquid nitrogen. Total RNA was extracted using an RNeasy plant mini kit (Qiagen, http://www.qiagen.com ). Crude RNA preparations were treated with 10 units of RNase-free DNase I ( http://www.promega.com ), and the samples were purified according to the RNeasy plant mini kit protocol. cDNA was synthesized from 1.5 μg of DNA-free RNA template using an oligo(dT) primer and SuperScript II reverse transcriptase ( http://www.invitrogen.com ). RT-qPCR analysis was performed on an optical 96-well plate using SYBR Green PCR master mix (Applied Biosystems, http://www.appliedbiosystems.com ) and an ABI PRISM 7500 real-time PCR system (http://www.appliedbiosystems.com). The thermal cycle used was 95 °C for 15 min, followed by 40 cycles of 95 °C for 15 s, 60 °C for 30 s and 72 °C for 35 s. Specific primer pairs for each gene were designed using Beacon Designer 7.0 ( http://www.premierbiosoft.com ) and are listed in Supplementary Table 1 . Actin8 (At1g49240), UBC (At5g25760) and IPP2 (At3g02780) were used to normalize the expression levels and then standardized to the wild type under white light. Microarrays and data analysis The microarray experiment consisted in a factorial design comprising two genotypes (Col and bbx24-1 ) and two light treatments (white light and simulated shade). RNA material was extracted from 7-day-old seedlings. Two replicates per treatment were performed using Affymetrix Arabidopsis ATH1 GeneChip ( http://www.affymetrix.com ). RNA was prepared, labelled and hybridized in accordance with the manufacturer’s instructions. Data were normalized by multiplying the value of each gene by the mean of each chip, divided by the average intensity of all mean values. Significantly differentially expressed genes were identified by performing profile analysis using Significance Analysis of Microarrays with a δ -value of 1.40, which corresponds to a false-discovery rate of 4.12% (ref. 48 ). Genes with ‘absent’ calls and a signal of <50 units in all replicate experiments were filtered out. A test filter was performed to work only with those genes for which the ratio of expression showed at least a 1.5-fold change between Col and bbx24-1 . Clusters were generated using DNA-Chip Analyzer ( http://www.dchip.org ). Gene Ontology enrichment were analysed using the Classification SuperViewer Tool of the Bio-Array Resource ( http://bar.utoronto.ca ). A ranking score is calculated for each functional class. The input set is bootstrapped 100 times to provide some idea as to over- or under-representation reliability. Upstream promoter sequences (1,000 bp) of differentially expressed genes were analysed using Promoter at BAR ( http://bar.utoronto.ca ). The P value was determined using the hypergeometric probability distribution to find the likelihood of the observed number of elements occurring in a randomly chosen set of promoters ( P <0.05). Statistical significance of the overlap between two groups of genes was calculated as the representation factor, which is the number of overlapping genes divided by the expected number of overlapping genes estimated from two independent groups ( http://elegans.uky.edu/ ). Protein–protein interaction assays A pENTR vector carrying the coding sequence (CDS) of BBX24 was created by cloning BBX24 CDS into pCR8-GW vector (Invitrogen). Deleted versions of BBX24 were amplified by PCR and cloned into pCR8-GW/TOPO ( http://www.invitrogen.com ) to create pENTR vectors. Deletions of GAI are described in Gallego-Bartolomé et al . [49] The full-length BBX24 CDS was cloned into both pDEST22 and pDEST32, whereas deletions were cloned into pDEST22. Final bait and prey constructs were used to co-transform the yeast strain AH109 ( http://www.clontech.com ). Yeasts were selected in SD/-Leu/-Trp/-His and with different amounts of 3-aminotriazol ( http://www.sigmaaldrich.com ) to test interactions. Primers used for cloning are listed in Supplementary Table 1 . For BiFC, GAI and BBX24 CDSs were transferred into pMDC43-YFC and pMDC43-YFN vectors, respectively [50] . To study the interference of BBX24 in the interaction between GAI and PIF4, the GAI and PIF4 CDSs were transferred to pMDC43-YFC and pMDC43-YFN vectors, respectively, whereas that of BBX24 was transferred to pEarleyGate-201(ref. 47 ) to create a HA fusion. BiFC analysis was performed as described in Locascio et al . [15] . The oligonucleotides used as primers to detect GAI , PIF4 and EF1-α from N. benthamiana leaves by RT-sqPCR have been described [38] , [51] . For co-immunoprecipitation assays in Nicotiana benthamiana , BBX24 CDS was transferred as indicated above into pEarleyGate-104 (ref. 47 ) to create the YFP-BBX24 fusion. RFP-GAI is described in Locascio et al . [15] Each construct was introduced into Agrobacterium tumefaciens C58 cells. Three days after infiltration, leaves were collected and frozen in liquid nitrogen. Infiltrated tissues were ground and homogenized in two volumes of cold extraction buffer (50 mM Tris·HCl (pH 7.5), 50 mM NaCl, 1% (vol/vol) Nonidet P-40 and 1 × complete protease inhibitor mixture ( http://www.roche.com )). Extracts were centrifuged twice for 30 min at 16,000 × g in a top bench microcentrifuge at 4 °C. Total soluble proteins in the supernatant were quantified by Bradford’s assay. Ten micrograms of soluble proteins were saved to be used as input, and the remaining proteins were incubated with 50 μl of anti-GFP paramagnetic MicroBeads ( https://www.miltenyibiotec.com ) on ice for 2 h in a total volume of 1 ml. Extracts were loaded at room temperature onto μ-columns ( https://www.miltenyibiotec.com ) previously equilibrated with extraction buffer. Columns were kept at room temperature and washed four times with 200 μl of cold extraction buffer and once with 100 μl of cold washing buffer 2 (20 mM Tris·HCl, pH 7.5) supplied in the kit ( https://www.miltenyibiotec.com ). Proteins were eluted in 50 μl of denaturing elution buffer following the manufacturer’s instructions. Immunoprecipitated proteins were run in 12% SDS-polyacrylamide gel electrophoresis, immunoblotted and detected with anti-GAI antibody diluted 1:1,000 (ref. 52 ). Subsequently, blots were stripped out and incubated with anti-GFP antibody diluted 1:1,000 (Ab290; https://www.abcam.com ). The western blot in Fig. 7b was incubated with an anti-RGA antibody diluted 1:300 ( http://www.agrisera.com ). Reporter constructs and transcriptional assays pPIL1::LUC reporter constructs are describe in Zhang et al . [31] As effector proteins, we used PIF4-YFP, BBX24-HA and GAI-GFP fusions [15] . To generate PIF4-YFP fusion, the pENTR carrying PIF4 CDS from REGIA (Regulatory Gene Initiative in Arabidopsis [53] ) was recombined by LR reaction into a pEarleyGate-104 (ref. 47 ). BBX24-HA construct was made by recombining the pENTR carrying BBX24 into the vector pEarleyGate-201 by the LR reaction. Transient expression in leaves of 4-week-old N. benthamiana was done by the infiltration mixture. To prevent silencing, A. tumefaciens C58 carrying a construct that expresses the silencing suppressor P19 was included in the mixtures. The ratio of cells carrying P19:reporter:effector constructs was 1:1:1 for PIF4 and BBX24, whereas it was 1:1:4 for GAI. Mixtures were incubated for 3 h in darkness at RT before infiltration. Firefly and the control Renilla–LUC activities were assayed from leaf extracts collected 3 days after infiltration with the Dual-Glo Luciferase Assay System (Promega) and quantified with a GloMax 96 Microplate Luminometer (Promega). Accession codes: microarray data associated with this study has been deposited in the NCBI GEO database under the accession code GSE 64755 . How to cite this article: Crocco, C. D. et al . The transcriptional regulator BBX24 impairs DELLA activity to promote shade avoidance in Arabidopsis thaliana . Nat. Commun. 6:6202 doi: 10.1038/ncomms7202 (2015).